A histone H3K36 chromatin switch coordinates DNA double-strand break repair pathway choice DNA double-strand break (DSB) repair is a highly regulated process performed predominantly by non-homologous end joining (NHEJ) or homologous recombination (HR) pathways. How these pathways are coordinated in the context of chromatin is unclear. Here we uncover a role for histone H3K36 modification in regulating DSB repair pathway choice in fission yeast. We find Set2-dependent H3K36 methylation reduces chromatin accessibility, reduces resection and promotes NHEJ, while antagonistic Gcn5-dependent H3K36 acetylation increases chromatin accessibility, increases resection and promotes HR. Accordingly, loss of Set2 increases H3K36Ac, chromatin accessibility and resection, while Gcn5 loss results in the opposite phenotypes following DSB induction. Further, H3K36 modification is cell cycle regulated with Set2-dependent H3K36 methylation peaking in G1 when NHEJ occurs, while Gcn5-dependent H3K36 acetylation peaks in S/G2 when HR prevails. These findings support an H3K36 chromatin switch in regulating DSB repair pathway choice. DNA double-strand breaks (DSBs) if unrepaired or inappropriately repaired can lead to cell death or genomic instability [1] . To prevent such undesirable outcomes, cells employ the evolutionarily conserved non-homologous end joining (NHEJ) or homologous recombination (HR) repair pathways to restore genome integrity. During NHEJ, the broken ends are protected by the Ku70/80 heterodimer, which in mammalian cells facilitates recruitment of the DNA-dependent protein kinase (DNA-PKcs). This facilitates processing of damaged DNA ends and subsequent ligation of the compatible ends through the activity of the conserved DNA ligase 4, XLF, XRCC4 complex [2] . HR is initiated by resection of the 5′ end of the DSB to generate a 3′ single-stranded DNA (ssDNA) overhang. This is bound by replication protein A (RPA), and, during mitotic recombination, a Rad51 nucleofilament is formed promoting strand invasion of the sister chromatid or homologous chromosome, which is used as a repair template before second end capture [3] . DSB repair pathway choice is influenced by a number of factors including cell cycle phase. In yeast, NHEJ is restricted to G1, while HR operates in S and G2 phase cells when a sister chromatid is available as a repair template [4] , [5] , [6] . DSB resection is a critical determinant of repair pathway choice and is highly regulated as inappropriate pathway deployment can result in pathological consequences [1] . Here we have investigated the role of histone H3 lysine 36 (H3K36) modification in DSB repair pathway choice. H3K36 methylation is associated with numerous functions [7] . In Saccharomyces cerevisiae , SET ( S u(var)3-9, E z, T rithorax ) domain-containing 2 (Set2) is responsible for mono, di and trimethylation of H3K36 (ref. 8 ). In humans, H3K36 methylation is catalysed through the activities of eight distinct enzymes, while SETD2/HYPB uniquely catalyses the trimethylation of H3K36 (ref. 9 ). Importantly, SETD2 has recently been classified as a novel tumour suppressor, suggesting a role in genome stability [10] , [11] , [12] , [13] , [14] . Links between histone H3K36 methylation and DSB repair have been identified in yeast and human cells [15] , [16] , [17] . These findings support a role for H3K36 methylation in promoting efficient NHEJ, although the molecular basis of this is unknown. A role for H3K36 methylation in promoting HR has also been recently described [18] . Histone H3K36 residues can also be acetylated, which in S. cerevisiae is performed by the Gcn5 histone acetyltransferase (HAT) [19] . Gcn5 is the catalytic subunit of the SAGA, ADA and SLIK chromatin-modifying complexes that post-translationally modify histones and regulate gene expression [20] . Gcn5 has also been associated with DSB repair in yeast and human cells, and these data suggest a possible role in HR [21] , [22] , [23] , [24] . Structurally, H3K36 residues can be either methylated or acetylated raising the intriguing possibility that these exclusive marks might drive distinct biological effects within chromatin [19] . As NHEJ and HR pathways can exhibit an antagonistic relationship [25] , [26] , we have investigated the functional interplay between these H3K36 modifications in regulating DSB repair pathway choice in fission yeast. Here we identify a role for Set2-dependent H3K36 methylation in facilitating NHEJ. In contrast, we find Gcn5-dependent H3K36 acetylation promotes HR. Together our findings support a role for an H3K36 chromatin switch in coordinating DSB repair pathway choice in fission yeast. Set2 methyltransferase suppresses homologous recombination To determine a possible role for H3K36 modification in DSB repair, we examined the effect of deleting Set2 on damage sensitivity. set2 Δ cells was found to exhibit modest sensitivity to both the radiomimetic bleomycin and ionizing radiation (IR) compared with wild-type cells, indicating a role for Set2 in the cellular response to DSBs ( Fig. 1a,b ). To investigate the role of Set2 methyltransferase activity in the DNA damage response, a highly conserved arginine within the catalytic SET domain was mutated to glycine ( set2-R255G ) within the endogenous set2 + gene, which was predicted to disrupt the methyltransferase activity ( Fig. 1c ) [8] , [27] . No H3K36me3 was observed in set2 Δ cells, indicating an absolute requirement for Set2 in H3K36 trimethylation in fission yeast, as previously described [28] ( Fig. 1d ). Substantially reduced levels of H3K36me3 were observed in the set2-R255G mutant compared with wild type, indicating that this residue is required for optimal H3K36 methylation ( Fig. 1d ). To investigate a possible role for Set2 in DSB repair, we used a DSB assay to quantitate marker loss profiles and thus repair responses to a site-specific DSB within a non-essential minichromosome [29] ( Supplementary Fig. 1 ). This revealed that deletion of set2 + resulted in significantly elevated levels of gene conversion (GC) (72% P =0.02), compared with wild type (55%) ( Fig. 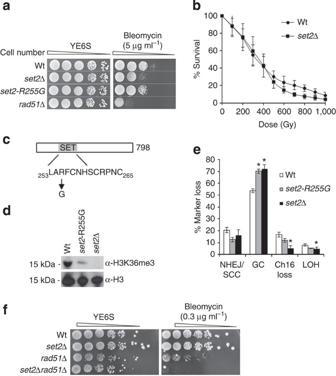Figure 1: Set2 is required to suppress HR and for resistance to DNA-damaging agents. (a) 10-fold serial dilutions of wild-type,set2Δ,set2-R255Gandrad51Δ strains on YE6S, YE6S+5 μg /ml bleomycin. Plates were incubated at 32 °C for 3 days. At least two biological replicates were performed. (b) IR survival curve for wild-type (Wt) andset2Δ strains. Means±s.e. of three experiments are shown. (c) A schematic of the structure of Set2 with SET (ASW) domain shown with amino-acid sequences indicating arginine residue mutated in SET domain of theset2-R255Gmutant. (d) Western blot analysis of H3K36me3 levels in wild-type (Wt),set2Δ andset2-R255Gcells. (e) Percentage DSB-induced marker loss in wild type (Wt),set2Δ andset2-R255Gcontaining Ch16-RMGAH. The levels of NHEJ/SCC, GC, Ch16loss and LOH are shown. Means±s.e. of three experiments are shown. * represents significant difference compared with wild-type (P<0.05,t-test). See alsoSupplementary Fig. 1andTable 1. (f)set2Δ cells are sensitive to bleomycin in combination withrad51Δ. Fivefold serial dilutions of wild-type (Wt),set2Δ,rad51Δ andset2Δrad51Δ cells were grown on YE6S and YE6S+0.3 μg /ml−1bleomycin. 1e and Table 1 ). HO induction in a set2-R255G background resulted in a very similar DSB repair profile to set2 Δ with significantly elevated levels of GC (70% P <0.01), compared with wild type ( Fig. 1e and Table 1 ), thus identifying a role for Set2 methyltransferase activity in suppressing HR repair. Consistent with an HR-independent role for Set2 in DSB repair, a double mutant set2 Δ rad51 Δ exhibited acute sensitivity to bleomycin compared with the single mutants ( Fig. 1f ), indicating that Set2 is required for survival in the absence of HR. Figure 1: Set2 is required to suppress HR and for resistance to DNA-damaging agents. ( a ) 10-fold serial dilutions of wild-type, set2Δ , set2-R255G and rad51 Δ strains on YE6S, YE6S+5 μg /ml bleomycin. Plates were incubated at 32 °C for 3 days. At least two biological replicates were performed. ( b ) IR survival curve for wild-type (Wt) and set2 Δ strains. Means±s.e. of three experiments are shown. ( c ) A schematic of the structure of Set2 with SET (ASW) domain shown with amino-acid sequences indicating arginine residue mutated in SET domain of the set2-R255G mutant. ( d ) Western blot analysis of H3K36me3 levels in wild-type (Wt), set2 Δ and set2-R255G cells. ( e ) Percentage DSB-induced marker loss in wild type (Wt), set2 Δ and set2-R255G containing Ch 16 -RMGAH. The levels of NHEJ/SCC, GC, Ch 16 loss and LOH are shown. Means±s.e. of three experiments are shown. * represents significant difference compared with wild-type ( P <0.05, t -test). See also Supplementary Fig. 1 and Table 1 . ( f ) set2 Δ cells are sensitive to bleomycin in combination with rad51 Δ. Fivefold serial dilutions of wild-type (Wt), set2 Δ, rad51 Δ and set2 Δ rad51 Δ cells were grown on YE6S and YE6S+0.3 μg /ml −1 bleomycin. Full size image Table 1 Analysis of DSB repair outcomes in different genetic backgrounds. Full size table Set2 methyltransferase is required for canonical NHEJ As HR and NHEJ can compete during DSB repair [25] , [26] , the increased HR observed in the set2 Δ and set2-R255G backgrounds could have arisen from reduced NHEJ, which may have been masked by sister chromatid conversion (SCC) in our DSB assay ( Supplementary Fig. 1 ). Consistent with a role for Set2 in NHEJ, lig4 Δ was found to be epistatic with set2 Δ in response to bleomycin ( Fig. 2a ). Further, quantitating colony survival indicated that the set2 Δ lig4 Δ double mutant phenocopied the sensitivity of set2 Δ to bleocin ( Fig. 2b ). These data support a role for Set2 in canonical NHEJ. However, as set2 Δ was more sensitive than lig4 Δ, Set2 must also perform an additional NHEJ-independent function in response to DNA damage. The ability of Set2 to repair a DSB by NHEJ was further assessed using a plasmid-rejoining assay, in which recircularization of linearized LEU2 plasmids by NHEJ allows stable propagation of leu + colonies. LEU2 plasmids linearized with PstI (3′ overhang), EcoRI (5′ overhang) or PvuII (blunt) were transformed into wild-type, lig4 Δ, and set2 Δ cells and the number of leu + colonies quantified. Plasmid rejoining was impaired in set2 Δ cells compared with wild-type cells ( Fig. 2c ). Plasmid rejoining was also impaired in the set2-R255G strain ( Supplementary Fig. 2 ). These results together define a role for Set2 methyltransferase activity in promoting canonical NHEJ and are consistent with impaired NHEJ in set2 Δ cells leading to increased HR. No significant changes in gene expression of NHEJ or HR repair genes were observed in set2 Δ cells in the absence or presence of damage, suggesting a direct role in NHEJ. ( Supplementary Fig. 3a,b ). 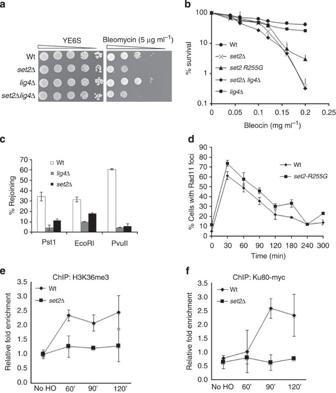Figure 2: Set2 is required for C-NHEJ. (a) Serial dilutions of the indicated strains were spotted onto YE6S containing 5 μg ml−1bleomycin or no drug. Plates were incubated at 32 °C for 3 days. (b) Percentage survival of strains indicated compared with wild-type following plating on YE6S +/− the indicated bleocin concentration. Plates were incubated for 3 days at 32 °C and then scored. Means±s.e. of four independent experiments are shown. (c) Set2 is required for NHEJ plasmid rejoining. The percentage of leu+colonies obtained following transformation rejoining of aLEU2plasmid (pAL19) linearized with EcoRI, PstI or PvuII following transformation into wild-type (Wt),lig4Δ andset2Δ strains compared with uncut plasmid control is shown. Means±s.e. of three experiments are shown. See alsoSupplementary Fig. 2. (d) Quantification of Rpa1(Rad11)-GFP foci in wild-type (Wt) andset2-R255Gstrains following exposure to 50 Gy IR treatment. Mean±s.e. of three experiments are shown. See alsoSupplementary Fig. 5. (e) DSB induction results in a Set2-dependent increase in histone H3K36me3 levels proximal to the HO break. qChIP enrichments of H3K36me3 in wild-type (Wt) orset2Δ cells at various times (60, 90 or 120 min) following urg-HO induced DSB induction at theMATasite between SPAC3H1.10 andhsr1on Chromosome I, as previously described59. Enrichment of immunoprecipitated DNA at 50 bp from the break relative to that atact1is presented, as a ratio of that observed in a strain expressing no HO endonuclease. Error bars represent s.d. from at least two biological replicates. (f) DSB induction results in a Set2-dependent increase in Ku80 levels proximal to the HO break. qChIP enrichments of Ku80-myc in wild-type (Wt) orset2Δ cells at various times (60, 90 or 120 min) following urg-HO induction as described above. Enrichment of immunoprecipitated DNA at 50 bp from the break, relative to that at thefbp1locus is presented. Error bars represent s.d. from at least two biological replicates. Figure 2: Set2 is required for C-NHEJ. ( a ) Serial dilutions of the indicated strains were spotted onto YE6S containing 5 μg ml −1 bleomycin or no drug. Plates were incubated at 32 °C for 3 days. ( b ) Percentage survival of strains indicated compared with wild-type following plating on YE6S +/− the indicated bleocin concentration. Plates were incubated for 3 days at 32 °C and then scored. Means±s.e. of four independent experiments are shown. ( c ) Set2 is required for NHEJ plasmid rejoining. The percentage of leu + colonies obtained following transformation rejoining of a LEU2 plasmid (pAL19) linearized with EcoRI, PstI or PvuII following transformation into wild-type (Wt), lig4 Δ and set2 Δ strains compared with uncut plasmid control is shown. Means±s.e. of three experiments are shown. See also Supplementary Fig. 2 . ( d ) Quantification of Rpa1(Rad11)-GFP foci in wild-type (Wt) and set2-R255G strains following exposure to 50 Gy IR treatment. Mean±s.e. of three experiments are shown. See also Supplementary Fig. 5 . ( e ) DSB induction results in a Set2-dependent increase in histone H3K36me3 levels proximal to the HO break. qChIP enrichments of H3K36me3 in wild-type (Wt) or set2 Δ cells at various times (60, 90 or 120 min) following urg-HO induced DSB induction at the MATa site between SPAC3H1.10 and hsr1 on Chromosome I, as previously described [59] . Enrichment of immunoprecipitated DNA at 50 bp from the break relative to that at act1 is presented, as a ratio of that observed in a strain expressing no HO endonuclease. Error bars represent s.d. from at least two biological replicates. ( f ) DSB induction results in a Set2-dependent increase in Ku80 levels proximal to the HO break. qChIP enrichments of Ku80-myc in wild-type (Wt) or set2 Δ cells at various times (60, 90 or 120 min) following urg-HO induction as described above. Enrichment of immunoprecipitated DNA at 50 bp from the break, relative to that at the fbp1 locus is presented. Error bars represent s.d. from at least two biological replicates. Full size image To determine the mechanism by which Set2 promotes NHEJ, we investigated whether H3K36me-interacting proteins (readers) functioned in NHEJ. In S. cerevisiae , co-transcriptional methylation of H3K36 by Set2 leads to recruitment of the Rpd3S HDAC complex, which deacetylates histones in the wake of elongating PolII [30] . However, analysis of alp13 Δ or clr6-1 , which disrupt the equivalent deacetylase complex in S. pombe [31] , [32] , failed to disrupt NHEJ ( Supplementary Fig. 4a,b ), indicating that Set2 functions independently of the Clr6 HDAC complex to promote NHEJ. To further investigate the role of Set2 in promoting NHEJ and suppressing HR, we considered a possible role for Set2 in protecting DSB ends from resection. To test this, levels of RPA foci were investigated following exposure to 50 Gy IR using a construct in which the large subunit of RPA was GFP-tagged (Rad11-GFP) [33] . As expected, loss of end-protection in ku70 Δ cells leads to increased Rad11-GFP foci following DSB induction [34] ( Supplementary Fig. 5 ). Similarly, an increase in Rad11-GFP foci was observed in a set2-R255G mutant background compared with wild type ( Fig. 2d ), suggesting a role for Set2 methyltransferase activity in preventing break-induced ssDNA formation analogously to Ku70, thus providing an explanation for the increase in HR in the absence of Set2. We also observed increased level of RPA levels in G1-arrested set2 Δ cells compared with G1-arrested wild-type cells ( Supplementary Fig. 6 ). We next investigated whether H3K36 methylation was induced in response to a site-specific DSB. Chromatin immunoprecipitation (ChIP) analysis revealed that H3K36me3 levels increase in a Set2-dependent manner following HO-induced DSB induction ( Fig. 2e ). Given the loss of end protection and increased HR observed following Set2 loss, we examined a possible role for Set2-dependent H3K36 methylation in Ku recruitment to a DSB. ChIP analysis revealed a significant reduction in the levels of Ku80-myc associated with a HO-induced DSB in a set2 Δ background ( Fig. 2f ). Together these findings support a role for Set2-dependent H3K36 methylation in Ku recruitment to break-sites thereby facilitating NHEJ. H3K36 methylation and acetylation are mutually inhibitory Lysine residues in proteins can be methylated or acetylated in a mutually exclusive manner. As loss of Set2 led to DSB end deprotection and increased HR, we investigated whether these events were associated with loss of H3K36 methylation and increased H3K36 acetylation. In budding yeast, H3K36 is acetylated by the Gcn5 histone acetyltransferase (HAT) [19] . To examine the relationship between H3K36 modifications, levels of H3K36 methylation and acetylation were analysed from nuclear extracts of wild-type, set2 Δ or gcn5 Δ cells by western blot analysis. In contrast to wild type, H3K36ac was undetectable in gcn5 Δ cells, thus defining an evolutionarily conserved role for Gcn5 as the H3K36 HAT in fission yeast, as in budding yeast ( Fig. 3a ) [19] . In the absence of Set2, H3K36ac levels were elevated compared with wild type ( Fig. 3a ). As expected, no H3K36me3 was observed in set2 Δ cells, consistent with Set2 being essential for H3K36 methylation ( Figs 1d and 3b ). Surprisingly, H3K36me3 levels in gcn5 Δ cells were much higher than that observed in wild-type cells ( Fig. 3b ). Thus, Gcn5-dependent H3K36ac inhibits H3K36me3, indicating that these H3K36 modifications are mutually inhibitory. 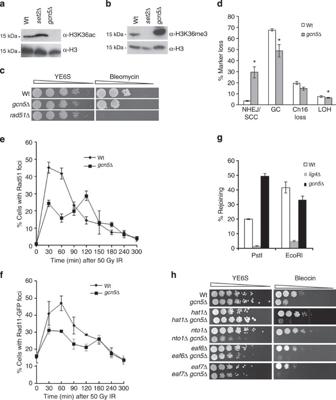Figure 3: Gcn5 promotes HR and suppresses NHEJ. (a,b) Methylation and acetylation of H3K36 are mutually inhibitory. (a) Western blot analysis of H3K36me3 in wild type (Wt),set2Δ andgcn5Δ nuclear extract. (b) Western blot analysis of H3K36ac in wild type (Wt),set2Δ andgcn5Δ nuclear extract. (c) Fivefold serial dilutions of wild-type (Wt),gcn5Δandrad51Δ strains on YE6S and YE6S+5 μg ml−1bleomycin. Plates were incubated at 32 °C for 3 days. At least two biological replicates were performed. (d) Percentage DSB-induced marker loss in wild type (Wt) andgcn5Δ containing Ch16-RMYAH. The levels of NHEJ/SCC, GC, Ch16loss and LOH are shown. Means±s.e. of three experiments are shown. * represents significant difference compared with wild type (P<0.05,t-test). See alsoTable 1. (e) Quantification of Rad51-CFP foci in wild-type andgcn5Δ strains following exposure to 50 Gy IR. (f) Quantification of Rpa1(Rad11)-GFP foci in wild-type andgcn5Δ strains strains following exposure to 50 Gy IR treatment. Data are the mean of three experiments and error bars (±s.e.) are shown. (g) Gcn5 suppresses NHEJ plasmid rejoining. The percentage of leu+colonies obtained following transformation and rejoining of aLEU2plasmid (pAL19) linearized with EcoRI, PstI into wild-type,lig4Δ andgcn5Δ strains compared with uncut plasmid control is shown. Means±s.e. of three experiments are shown. (h) Gcn5 functions redundantly with other HAT complex subunits in the DNA damage response. Fivefold serial dilutions of wild-type (Wt),gcn5Δ,hat1Δ, hat1Δgcn5Δ,nto1Δ,nto1Δgcn5Δ,eaf6Δ, eaf6Δgcn5Δ,eaf7Δ, andeaf7Δgcn5Δ strains on YE6S and YE6S+5 μg ml−1bleocin. At least two biological replicates were performed. Figure 3: Gcn5 promotes HR and suppresses NHEJ. ( a , b ) Methylation and acetylation of H3K36 are mutually inhibitory. ( a ) Western blot analysis of H3K36me3 in wild type (Wt), set2 Δ and gcn5 Δ nuclear extract. ( b ) Western blot analysis of H3K36ac in wild type (Wt), set2 Δ and gcn5 Δ nuclear extract. ( c ) Fivefold serial dilutions of wild-type (Wt), gcn5Δ and rad51 Δ strains on YE6S and YE6S+5 μg ml −1 bleomycin. Plates were incubated at 32 °C for 3 days. At least two biological replicates were performed. ( d ) Percentage DSB-induced marker loss in wild type (Wt) and gcn5 Δ containing Ch 16 -RMYAH. The levels of NHEJ/SCC, GC, Ch 16 loss and LOH are shown. Means±s.e. of three experiments are shown. * represents significant difference compared with wild type ( P <0.05, t -test). See also Table 1 . ( e ) Quantification of Rad51-CFP foci in wild-type and gcn5 Δ strains following exposure to 50 Gy IR. ( f ) Quantification of Rpa1(Rad11)-GFP foci in wild-type and gcn5 Δ strains strains following exposure to 50 Gy IR treatment. Data are the mean of three experiments and error bars (±s.e.) are shown. ( g ) Gcn5 suppresses NHEJ plasmid rejoining. The percentage of leu + colonies obtained following transformation and rejoining of a LEU2 plasmid (pAL19) linearized with EcoRI, PstI into wild-type, lig4 Δ and gcn5 Δ strains compared with uncut plasmid control is shown. Means±s.e. of three experiments are shown. ( h ) Gcn5 functions redundantly with other HAT complex subunits in the DNA damage response. Fivefold serial dilutions of wild-type (Wt), gcn5 Δ, hat1 Δ , hat1 Δ gcn5 Δ, nto1 Δ, nto1 Δ gcn5 Δ, eaf6 Δ , eaf6 Δ gcn5 Δ, eaf7 Δ, and eaf7 Δ gcn5 Δ strains on YE6S and YE6S+5 μg ml −1 bleocin. At least two biological replicates were performed. Full size image Gcn5 promotes HR and suppresses NHEJ As Gcn5-dependent H3K36ac inhibits Set2-dependent H3K36me, which our data indicate is required for NHEJ, we investigated whether Gcn5 facilitated HR repair. We found that gcn5 Δ cells exhibited mild sensitivity to bleomycin ( Fig. 3c ) consistent with a role for Gcn5 in DSB repair [35] . Microarray analysis previously performed on gcn5 Δ cells did not identify any alteration in the transcription of DSB repair genes [36] , suggesting a direct role for Gcn5 in DSB repair. Therefore, a role for Gcn5 in DSB repair was further examined using the DSB assay ( Supplementary Fig. 1 ). DSB induction in a gcn5 Δ background resulted in significantly increased levels of NHEJ/SCC (33%, P <0.01) and significantly reduced GC (45%, P <0.01) compared with wild-type cells ( Fig. 3d and Table 1 ). These results identified a role for Gcn5 in promoting efficient HR. Further, these results contrasted with those observed following loss of Set2 methyltransferase. To investigate when Gcn5 acts during HR, the kinetics of Rad51-CFP foci were analysed in gcn5 Δ cells following treatment with IR. gcn5 Δ cells exhibited a striking reduction in Rad51-CFP foci 30–60 min following treatment with 50 Gy IR, compared with wild-type cells ( Fig. 3e ). Following this initial decline, the percentage of cells with Rad51-CFP foci increased again 120 min after damage. Importantly, Rad51-CFP expression was not affected in gcn5 Δ cells ( Supplementary Fig. 7 ). These data indicated that gcn5 Δ cells, although still able to recruit Rad51, did so much less effectively than wild-type cells, indicating a role for Gcn5 in HR before strand invasion (synapsis). To further address the presynaptic role of Gcn5, the recruitment of RPA subunit Rad11-GFP to ssDNA following exposure to 50 Gy IR was examined. In contrast to wild-type cells, the levels of Rad11-GFP foci were reduced in gcn5 Δ cells at earlier time points ( Fig. 3f ). Therefore, Gcn5 functions presynaptically during HR to promote ssDNA formation following DSB induction. We noted that again, Gcn5 loss exhibited an opposite phenotype to that observed in a set2-R255G background ( Fig. 2d ). Given the reduced ssDNA formation following DSB induction, we further addressed whether DSB repair was associated with elevated levels of NHEJ in a gcn5 Δ background. To confirm whether NHEJ was increased following DSB induction in the gcn5 Δ mutant ( Fig. 3d ), repair in a gcn5 Δ lig4 Δ double mutant was assessed using the DSB assay ( Supplementary Fig. 1 ). The proportion of NHEJ/SCC colonies was reduced in a gcn5 Δ lig4 Δ background (23%) compared with gcn5 Δ (33%) consistent with 10% of this population being attributable to NHEJ in a gcn5 Δ strain ( Table 1 ). This level is significantly greater than the NHEJ/SCC level in wild-type cells (4% P <0.01), and thus represents a significant increase in NHEJ in the gcn5 Δ mutant. A similar profile was observed in a gcn5 Δ set2 Δ double mutant ( Table 1 ). Further analysis by the plasmid-rejoining assay indicated that gcn5 Δ cells exhibited consistently increased rejoining of a Pst I linearized plasmid compared to wild-type cells, although this appeared to depend on the presence of a 3′ overhang, as the same was not observed for an EcoRI-linearized plasmid ( Fig. 3g ). As gcn5 Δ exhibited mild sensitivity to DNA damage compared with rad51 Δ ( Fig. 3c ), we tested whether Gcn5 functioned redundantly with other HAT complexes to facilitate the DNA damage response. We found that deletion of gcn5 + together with genes encoding the histone acetyltransferase Hat1 (ref. 37) [37] , Nto1 (a subunit of the NuA3/Mst2 complex) [35] , Eaf6 (a subunit of both NuA3 and NuA4) [35] or Eaf7 (a subunit of the NuA4 complex) [38] resulted in a striking increase in bleocin sensitivity compared with the single mutants ( Fig. 3h ). These findings support a key role for Gcn5 in facilitating the DNA damage response in conjunction with other HAT complexes. These findings are consistent with and extend previous observations [35] , [37] , [39] . Role for H3K36 modification in DSB repair To test the role of H3K36 modification in DSB repair, we tested the sensitivity of an H3K36R mutant to DSB-inducing agents. No H3K36me3 was detected in H3K36R cells ( Fig. 4a ). The H3K36R mutant exhibited increased sensitivity to bleomycin ( Fig. 4b ) compared with wild-type or control cells ( H3.1 Δ H3.3 Δ) that retained an intact copy of the H3.2 gene. H3K36R mutant cells were elongated after 6 h exposure to bleomycin, in contrast to wild-type cells, consistent with a checkpoint-dependent cell cycle delay resulting from failed DSB repair ( Fig. 4c ). Further, the H3K36R mutant exhibited increased IR sensitivity compared with wild-type or H3.1 Δ H3.3 Δ controls ( Fig. 4d ). In addition, the H3K36R mutation did not affect total histone H3 levels ( Supplementary Fig. 8 ). These findings are in accordance with a role for H3K36 modification in DSB repair. 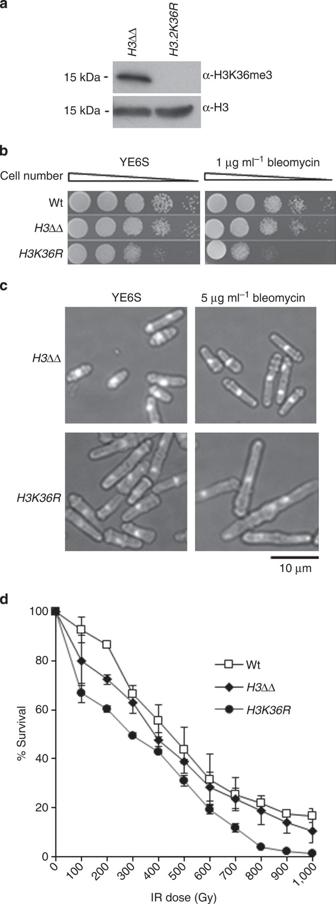Figure 4: Histone H3K36 is required for survival following exposure to DSB-inducing agents. (a) Western blot analysis of H3K36me3 in wild-type (Wt) andH3.2K36R H3.1ΔH3.3Δ (H3K36R)cells. α-H3 is shown as a loading control. (b) 10-fold serial dilutions of wild-type (Wt),H3ΔΔ andH3K36Rcells on YE6S, YE6S+1 μg ml−1bleomycin. Plates were incubated at 32 °C for 3 days. (c) Methanol-fixed asynchronous wild-type (Wt) andH3K36Rcells imaged following growth in the presence or absence of 5 μg ml−1bleomycin for 6 h. Bar, 10 μm. (d) IR survival curve for wild-type (Wt) andH3K36Rcells. Data are the mean of three experiments and error bars (±s.e.) are shown. Figure 4: Histone H3K36 is required for survival following exposure to DSB-inducing agents. ( a ) Western blot analysis of H3K36me3 in wild-type (Wt) and H3.2K36R H3.1 Δ H3.3 Δ ( H3K36R) cells. α-H3 is shown as a loading control. ( b ) 10-fold serial dilutions of wild-type (Wt), H3 ΔΔ and H3K36R cells on YE6S, YE6S+1 μg ml −1 bleomycin. Plates were incubated at 32 °C for 3 days. ( c ) Methanol-fixed asynchronous wild-type (Wt) and H3K36R cells imaged following growth in the presence or absence of 5 μg ml −1 bleomycin for 6 h. Bar, 10 μm. ( d ) IR survival curve for wild-type (Wt) and H3K36R cells. Data are the mean of three experiments and error bars (±s.e.) are shown. Full size image H3K36 modification and chromatin accessibility To address how H3K36 modification might affect DSB repair, we probed chromatin accessibility. Lysine acetylation neutralizes the positive charge on histones and thus weakens interactions between histones and DNA. Thus, more open chromatin arising from lysine acetylation may facilitate resection and subsequent DSB repair by HR. Conversely, lysine methylation might compact chromatin thereby inhibiting resection and promoting NHEJ. We therefore tested the global effect of deleting set2 + or gcn5 + on chromatin accessibility to micrococcal nuclease (MNase) following exposure to bleocin, as previously described [35] . We used the percentage of DNA that has a low molecular weight DNA (<tetranucleosome, ~600 bp) as a measure of chromatin accessibility. Deleting set2 + resulted in an increase in the level of low molecular weight DNA fragments, consistent with increased chromatin accessibility following DNA damage. In contrast, deleting gcn5 + resulted in reduced levels of MNase fragments of 600 bp or less, consistent with reduced chromatin accessibility in response to DNA damage ( Fig. 5a–c ). No obvious difference in DNA accessibility was observed in wild-type, set2 Δ or gcn5 Δ backgrounds in the absence of DNA damage ( Fig. 5d ). These findings are consistent with Set2 and Gcn5 regulating DSB repair pathway choice through modulating H3K36 methylation/acetylation status and subsequently chromatin accessibility to DSB repair factors. 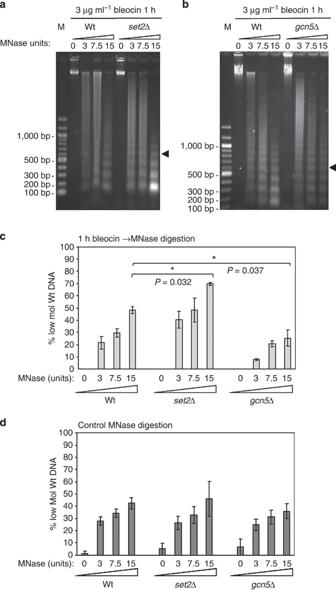Figure 5: Chromatin is more accessible to MNase following DNA damage inset2Δ cells and less accessible ingcn5Δ cells. (a,b) Mid-log phase cells were incubated in 3 μg ml−1bleocin for 1 h followed by MNase digestion for 10 min at the indicated concentrations. Digested chromatin DNA was resolved by gel electrophoresis and detected by ethidium bromide staining. The gels are representative of three independent repeats. (c) MNase digested chromatin DNA resolved on agarose gels were analyzed using Image J. The proportion of low molecular weight DNA (<tetranucleosome) was calculated as a percentage of the total sample.set2Δ cells have a significantly higher proportion of low molecular weight particles following digestion with 15U MNase (P=0.032;t-test), whilegcn5Δ cells have a significantly lower population of low molecular weight particles when compared with wild type (P=0.037;t-test), indicating an increase inset2Δ and a decrease ingcn5Δ chromatin accessibility. Data are the mean of at least three independent repeats and error bars (±s.e.) are shown (* denotesP<0.05;t-test). (d) Control MNase digestions (no bleocin treatment) were analysed as described forc. Data are the mean of at least three independent repeats and error bars (±s.e.) are shown. Comparison ofset2Δ andgcn5Δ samples with wild-type revealed no significant change in the proportion of low molecular weight particles (P-value cutoff 0.05;t-test). Figure 5: Chromatin is more accessible to MNase following DNA damage in set2 Δ cells and less accessible in gcn5 Δ cells. ( a , b ) Mid-log phase cells were incubated in 3 μg ml −1 bleocin for 1 h followed by MNase digestion for 10 min at the indicated concentrations. Digested chromatin DNA was resolved by gel electrophoresis and detected by ethidium bromide staining. The gels are representative of three independent repeats. ( c ) MNase digested chromatin DNA resolved on agarose gels were analyzed using Image J. The proportion of low molecular weight DNA (<tetranucleosome) was calculated as a percentage of the total sample. set2 Δ cells have a significantly higher proportion of low molecular weight particles following digestion with 15U MNase ( P =0.032; t -test), while gcn5 Δ cells have a significantly lower population of low molecular weight particles when compared with wild type ( P =0.037; t -test), indicating an increase in set2 Δ and a decrease in gcn5 Δ chromatin accessibility. Data are the mean of at least three independent repeats and error bars (±s.e.) are shown (* denotes P <0.05; t -test). ( d ) Control MNase digestions (no bleocin treatment) were analysed as described for c . Data are the mean of at least three independent repeats and error bars (±s.e.) are shown. Comparison of set2 Δ and gcn5 Δ samples with wild-type revealed no significant change in the proportion of low molecular weight particles ( P -value cutoff 0.05; t -test). Full size image H3K36 modification is cell cycle regulated In fission yeast, DSB repair pathway choice is cell cycle regulated, with NHEJ being utilized during G1, while HR is employed in S and G2 phases [6] . This prompted us to investigate whether H3K36 modification was cell cycle regulated. Following arrest in G1 by nitrogen starvation and release into the cell cycle ( Fig. 6a ), levels of chromatin bound H3K36 methylation and acetylation were determined by western blot. Cells with an increased 1C DNA content exhibited strikingly high H3K36me3 levels, while H3K36ac levels were low ( Fig. 6a,b ). Cell cycle progression resulted in a significant reduction in H3K36me3 levels after 2 h, whereas levels of H3K36me2 and H3K36me1 increased, consistent with S-phase progression ( Fig. 6a ). H3K36ac levels also increased with progression through S-phase, peaking at 5 h when the majority of cells were in G2 ( Fig. 6b ). These results indicate that modification of the H3K36 residue is cell cycle regulated. Further, the peak of methylation in a 1C population and acetylation in S/G2 is consistent with Set2-dependent H3K36 methylation being required for NHEJ, and Gcn5-dependent H3K36 acetylation being required for HR. The protein levels of Set2-myc and Gcn5-myc are constant during the cell cycle ( Supplementary Fig. 9 ). 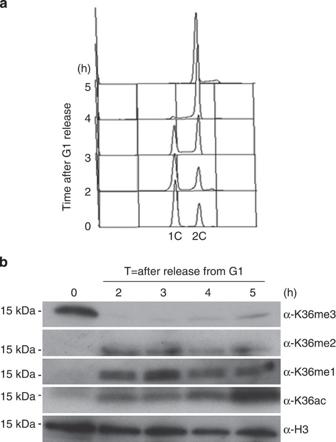Figure 6: H3K36 methylation and acetylation are cell cycle regulated. (a) Flow cytometry analysis of wild-type cells following release from nitrogen starvation. The data shown were performed from at least two biological replicates. (b) Acid-extracted histones prepared from a wild-type strain were resolved on a 4–20% SDS-PAGE gel, transferred to a PVDF membrane and probed for H3K36me3, H3K36me1 and H3K36ac. α-H3 is shown as a loading control. Western blot analysis of H3K36me3, H3K36me2, H3K36me1 and H3K36Ac in wild-type nuclear extract at the times shown following release from nitrogen starvation. Figure 6: H3K36 methylation and acetylation are cell cycle regulated. ( a ) Flow cytometry analysis of wild-type cells following release from nitrogen starvation. The data shown were performed from at least two biological replicates. ( b ) Acid-extracted histones prepared from a wild-type strain were resolved on a 4–20% SDS-PAGE gel, transferred to a PVDF membrane and probed for H3K36me3, H3K36me1 and H3K36ac. α-H3 is shown as a loading control. Western blot analysis of H3K36me3, H3K36me2, H3K36me1 and H3K36Ac in wild-type nuclear extract at the times shown following release from nitrogen starvation. Full size image Our findings support an H3K36 modification-mediated switch in coordinating DSB repair pathway choice in fission yeast. We define roles for Set2-dependent H3K36 methylation in reducing chromatin accessibility, reducing DSB resection and promoting NHEJ through Ku recruitment. In contrast, Gcn5-dependent H3K36 acetylation increases chromatin accessibility, increases DSB resection and promotes HR. Accordingly, loss of Set2 results in increased Gcn5-dependent H3K36Ac, open chromatin, increased resection and increased HR, while loss of Gcn5 results in increased Set2-dependent H3K36me, closed chromatin, reduced resection and increased NHEJ. The role for H3K36 modification in coordinating DSB repair was further confirmed by the observation that H3K36R mutation was sensitive to bleomycin and IR. Moreover, we found H3K36 modification to be cell cycle regulated with chromatin-bound H3K36me3 peaking in G1 where NHEJ occurs while H3K36 acetylation peaked in S/G2 phase when HR predominates. Together these findings support an H3K36 chromatin switch in coordinating DSB repair pathway choice in fission yeast. How might a switch in chromatin states dictated by H3K36 coordinate DSB repair pathway choice? Here we consider two non-exclusive models suggested by these and other findings. In the first ‘recruitment’ model, Set2-dependent H3K36 methylation is required to recruit the Ku70-Ku80 heterodimer to the break-site thereby promoting NHEJ. In contrast, Gcn5-dependent H3K36 acetylation may be refractory to Ku recruitment and could instead function to recruit HR factors. In this respect, Set2 may promote Ku recruitment through potential readers of the H3K36me mark. However, we found that neither Clr6, the Rpd3 homologue, nor Alp13, a subunit of the Clr6 HDAC complex II, exhibited defects in NHEJ. Instead, alp13 Δ and the temperature-sensitive clr6-1 allele were acutely sensitive to bleomycin [31] , [32] , and the set2 Δ alp13 Δ double mutant exhibited increased sensitivity, thus indicating a distinct function for the HDAC complex II in the DSB response. Other currently unknown H3K36me readers may promote Ku recruitment. Alternatively, H3K36me may recruit Ku indirectly through other chromatin factors. In this respect, components of the RSC chromatin remodelling complex physically interact with Ku80, and RSC has previously been shown to be required for loading of Ku onto breaks [40] , [41] . However, it is possible that Ku, which has a strong affinity for duplex DNA ends in vitro [42] , binds DNA ends independently of chromatin or associated factors in vivo. In a second ‘chromatin accessibility’ model, the distinct H3K36 chromatin states control end resection at a break-site via chromatin accessibility. Here, Set2-dependent H3K36me is proposed to promote closed chromatin, protecting ends from resection, thereby facilitating Ku recruitment or retention, and NHEJ. In contrast, Gcn5-dependent H3K36Ac is proposed to promote open acetylated chromatin and/or increased histone exchange, thus facilitating resection, reducing Ku binding or recruitment, and thus increasing HR. Consistent with this model, Set2 has been shown to suppress histone H3 and H4 acetylation by preventing histone exchange during transcription in S. cerevisiae. Increased histone exchange in the absence of Set2 facilitates histone acetylation thereby leading to increased cryptic transcripts [43] , [44] . In the context of DSB repair, increased histone exchange may facilitate transient nucleosome removal or the dynamic incorporation of histone variants thereby facilitating resection at DSBs. Indeed, a recent study using budding yeast characterizing the impact of chromatin on in vitro resection found that efficient resection by Sgs1-Dna2 required nucleosome-free regions adjacent to the DSB, while resection by Exo1 was completely blocked by nucleosomes. Moreover, incorporation of the histone variant H2A.Z was found to enhance resection [45] . Thus, Set2 may promote NHEJ through reducing chromatin accessibility to the resection machinery. The increased levels of Gcn5-dependent H3K36ac and damage-induced nucleosome mobility in a set2 Δ background, together with increased ssDNA formation following IR leading to increased HR compared with wild-type, are consistent with such a model ( Fig. 7 ). 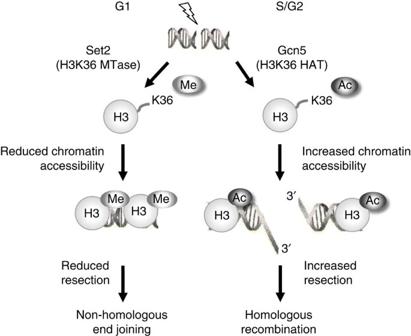Figure 7: An H3K36 chromatin switch regulates DSB repair pathway choice in fission yeast. In G1 high levels of Set2-dependent H3K36me (indicated) reduces nucleosome accessibility to repair factors, resulting in reduced resection and increased NHEJ repair of DSBs. In S/G2 high levels of Gcn5-dependent H3K36Ac (indicated) increases nucleosome accessibility to repair factors,resulting in increased resection and increased HR repair of DSBs. See text for details. Figure 7: An H3K36 chromatin switch regulates DSB repair pathway choice in fission yeast. In G1 high levels of Set2-dependent H3K36me (indicated) reduces nucleosome accessibility to repair factors, resulting in reduced resection and increased NHEJ repair of DSBs. In S/G2 high levels of Gcn5-dependent H3K36Ac (indicated) increases nucleosome accessibility to repair factors,resulting in increased resection and increased HR repair of DSBs. See text for details. Full size image Our findings support an early role for Gcn5-dependent H3K36Ac in facilitating HR. Loss of Gcn5 alone exhibited a modest sensitivity to DNA damaging agents; moreover, both Rad11 and Rad51 foci formation were delayed rather than abrogated in the absence of Gcn5. However, Gcn5 was found to play a critical role in the DNA damage response in conjunction with other HATs, including Hat1, NuA3 and NuA4, which have been previously associated with the DNA damage response and DSB repair [35] , [39] , [46] . Recently, recruitment of chromatin remodelling enzymes to a DSB was found to be dependent on the early steps of HR, while inhibited by NHEJ in budding yeast [47] . We speculate that Gcn5 may function early in HR in conjunction with other HATs to promote recruitment of ATP-dependent remodelers, repair factors and/or to increase DNA accessibility, thus promoting resection and HR. Importantly, H3K36 methylation is associated with DSB repair in other organisms. Indeed, roles for Set2-dependent H3K36 methylation in transcription-coupled DNA damage checkpoint activation in S. cerevisiae are reported in an accompanying manuscript [48] . Moreover, a H3K36 modification switch may help coordinate DSB repair pathway choice in humans. H3K36 dimethylation was reported to be increased at DSBs and to enhance NHEJ through recruiting NBS1 and Ku70 repair factors in a METNASE-dependent manner [17] . In contrast, a role for SETD2-dependent H3K36 trimethylation in facilitating HR in actively transcribed regions has recently been described [49] , [50] . Here, SETD2-dependent H3K36 trimethylation promotes HR through constitutive recruitment of Lens Epithelial Growth Factor p75 (LEDGF) to chromatin. In response to DNA damage, LEDGF recruits C-terminal binding protein interacting protein (CtIP), which promotes resection, thereby facilitating HR repair [18] . However, while LEDGF is present in higher eukaryotes, it is not evolutionarily conserved in budding or fission yeasts. Interestingly, Set1-dependent H3K4 methylation at DSBs also promotes NHEJ through Ku recruitment in budding yeast [51] . Thus, histone methylation plays an important role in facilitating NHEJ. How these methylation events are coordinated, and their functional antagonism through demethylation and acetylation is of considerable interest. The cell cycle regulation of H3K36 modification is surprising given the wide range of functions associated with H3K36 methylation. However, this finding is consistent with observations recently reported in human cells [52] and indicates that H3K36 cell cycle modification is evolutionarily conserved. How H3K36 modification is coordinated through the cell cycle and the functional implications for such regulation are currently unknown. The interplay between H3K36 acetylation and methylation has previously been proposed to regulate gene expression [19] . Here we show that this H3K36 chromatin switch helps to control DSB repair pathway choice in fission yeast. This chromatin switch, in concert with the complex networks that control DSB repair, ensures that the fidelity of the genome is maintained, preventing deleterious chromosomal rearrangements as a consequence of misuse of repair mechanisms. Yeast strains, media and genetic methods The strains used in this study are listed in Supplementary Tables 1 and 2 . Standard media and growth conditions were used throughout this work [53] . Cultures were grown in rich media (YE5S) or minimal media (EMM) at 32 °C with shaking, unless otherwise stated. Site-specific DSB assay Cells were grown exponentially in liquid culture for 48 h in the absence of thiamine (-T) to derepress HO endonuclease expression from the REP81X-HO plasmid. The percentage of colonies undergoing NHEJ/SCC (arg + Hyg R ade + his + ), gene conversion (arg + Hyg S ade + his + ), minichromosome loss (arg − Hyg S ade − his − ) or LOH (arg + Hyg S ade − his − ) was calculated (see also Supplementary Fig. 1 ). To determine levels of break-induced minichromosome loss, background minichromosome loss at 48 h in blank vector assays was subtracted from break-induced minichromosome loss at 48 h in cells transformed with pREP81X-HO. More than 1,000 colonies were scored for each time point, and each experiment was performed three times using three independently derived strains for all mutants tested. Fluorescent microscopy Asynchronous cultures were treated with +/− 5 μg ml −1 bleomycin (1 h 26 °C), before being fixed in methanol. Samples were rehydrated and stained with 4′,6-diamidino-2-phenylindole (DAPI) before examination using Zeiss Axioplan 2ie microscope, Hamamatsu Orca ER camera and micromanager software. For visualization of Rad11-GFP and Rad51-CFP foci, cells were irradiated with 50 Gy IR using a 137 Cs source with a dose rate of 2.8 Gy per minute, before being fixed and visualized as above. Serial dilution assay A dilution series for the indicated mutants was spotted onto YE6S plates and YE6S with the indicated concentration of MMS, bleomycin or bleocin. Plates were incubated at 32 °C for 2–3 days before analysis. Ionizing radiation survival curve Logarithmically growing cells were irradiated by using a 60 Co source at a dose rate of 31 Gy min −1 . Irradiated and unirradiated cells were plated on YE6S and incubated at 32 °C for 4 days before colonies were counted. Survival analysis Exponential cultures were obtained in liquid YE6S medium inoculated with a single colony picked from a freshly streaked (YE6S) stock plate and grown overnight at 32 °C with vigorous shaking. Cells were counted microscopically and only cultures with between 2 × 10 7 and 4 × 10 7 cells ml −1 were used. Cells were resuspended in YE6S at a density of 2 × 10 7 cells ml −1 , and serial dilutions were made and ~200 cells were plated on YE6S plates with the indicated dose of bleocin as well as an untreated control. Plates were incubated for 3 days at 32 °C and then scored. Quantitative chromatin immunoprecipitation (qChIP) Chromatin immunoprecipitation (ChIP) was performed as previously described [54] . In brief, cells were grown at 32 °C in Edinburgh Minimal Medium (EMM) supplemented with 0.25 mg/ml uracil, to induce Purg1 . One hundred millilitres of cells at O.D. 595 =0.4 were fixed in 1% formaldehyde (Sigma F8755-25ML) for 20 min at 24 °C with shaking. The reaction was quenched by adding 125 mM glycine for 5 min. Cells were lysed using a bead beater (Biospec Products), and cell lysates were sonicated in a Bioruptor (Diagenode) (15 min, 30 s On and 30 s Off at ‘High’ (200 W) position). For all ChIPs, 30 μl Protein G Dynabeads (Life Technologies) were used along with 3.5 μl ActiveMotif anti-H3K36me3 antibody (cat# 61101) or 1.5 μl anti-myc 9B11 (Cell Signaling), as appropriate. ChIPs were analysed by real-time PCR using Lightcycler 480 SYBR Green (Roche) with primers specific to the indicated regions. All ChIP enrichments were calculated as % DNA immunoprecipitated at the locus of interest (relative to the corresponding input samples) and normalized to % DNA immunoprecipitated at the act1 or fbp1 locus. Data averaged over at least two biological replicates are shown. Error bars represent s.d. values from at least two biological replicates. The primers used for qPCR analysis are listed in Supplementary Table 3 . Micrococcal nuclease digestion of chromatin One-hundred milliliters of cells were grown to mid-log phase in YE5S at 30 °C, treated with 3 μg ml −1 bleocin for 1 h, crosslinked with a final concentration of 1% formaldehyde (Sigma F8775) for 20 min at 30 °C and quenched by the addition of glycine to 125 mM. Cells were washed with CES buffer (50 mM citric acid/50 mM Na 2 HPO 4 (pH5.6), 40 mM EDTA (pH 8.0), 1.2 M sorbitol, 10 mM β-mercaptoethanol) and resuspended in 500 μl CES buffer with 0.5 mg Zymolyase-100T. Cells were spheroplasted by gentle shaking at 30 °C for up to 45 min, washed with ice cold 1.2 M sorbitol and resuspended in 800 μl NP-S buffer (1.2 M sorbitol, 10 mM CaCl 2 , 100 mM NaCl, 1 mM EDTA (pH 8.0), 14 mM β-mercaptoethanol, 50 mM Tris-HCl (pH 8.0), 0.075% NP-40, 5 mM spermidine, 0.1 mM PMSF, 1% Sigma protease inhibitor cocktail (Sigma P8215)). Spheroplasts were divided into four 200 μl aliquots, each mixed with 300 μl of NP-S buffer. MNase was added at the indicated concentrations, and samples were digested for 10 min at 37 °C. MNase activity was terminated by the addition of EDTA (pH 8.0) and SDS to the final concentrations of 50 mM and 0.2%, respectively. Samples were incubated at 65 °C overnight with 0.2 mg ml −1 proteinase K and 10 μg RNase A. DNA was subsequently purified by phenol:chloroform extraction followed by ethanol precipitation. Plasmid rejoining assay The plasmid rejoining assay was performed as previously described [55] . In brief, the cohesive-ended substrates for the NHEJ assay were prepared by excision of a ~500 bp PstI fragment or ~700 bp PvuII fragment from PS (p100) or a ~540 bp EcoRI fragment from PI (p101) followed by gel purification of the remaining linear vector. Logarithmically, growing cells (20 ml of OD595 0.5) were transformed with 1 μg of undigested control plasmid pAL19 or linear DNA using the lithium acetate method. As the plasmids contain a LEU2 marker, NHEJ frequency was calculated as the percentage of leu + colonies arising from cells transformed with linear plasmid over those transformed with undigested DNA. At least three experiments were performed for each strain, and the average percentage rejoining calculated. Microarray analysis Microarray analysis was performed as previously described [56] . In brief, Alexa 555- or 647-labelled cDNA was produced from the RNA, using a Superscript direct cDNA labelling system (Invitrogen) and Alexa 555 and 647 dUTP label mix. The cDNA was then purified using an Invitrogen PureLink PCR Purification system. The cDNA was hybridized to the array using a Gene Expression Hybridization kit (Agilent). The array was an Agilent custom-designed array containing 60-mer oligonucleotides synthesized in situ on the array and contained 4 × 44,000 probes. Following hybridization for at least 17 h, the array was washed using a Gene Expression Wash Buffer kit (Agilent) and scanned in an Agilent Array Scanner. The microarray signal was extracted using GenePix. Analysis of cell cycle-regulated histone modifications The wild-type yeast strain was arrested in G1 using nitrogen starvation [57] and released from the block. Samples were taken over a 5-h time course. The samples then underwent the histone acid-extraction method to purify histones for analysis by western blotting as previously described [58] . In brief, one litre of cells were collected by centrifugation. The cell pellet was resuspended in spheroplasting buffer (1.2 M Sorbitol, 20 mM Hepes pH 7.4, 1 mM PMSF, 0.5 μg ml −1 Leupeptin, 0.7 μg ml −1 Pepstatin) containing 10 mM dithiothreitol (DTT) and 2 mg ml −1 Zymolyase 20-T (MP Biomedicals) and then incubated in a 32 °C water bath until 90% of cells had lost their cell walls. Cells were centrifuged and resuspended in Nuclei Isolation Buffer (0.25 M Sucrose, 60 mM KCl, 14 mM NaCl, 5 mM MgCl 2 , 1 mM CaCl 2 , 15 mM MES, pH 6.6, 0.8% Triton X-100, 0.7 μg ml −1 Pepstatin, 1 mM PMSF, 0.5 μg ml −1 Leupeptin) on ice water for 20 min. After spinning and washing, most of the chromatin was in the pellet. Histones were extracted by resuspending the pellet in 10 ml of cold 0.4 N H 2 SO 4 . Protein extracts were made by TCA extraction and analysed by western blotting as previous described [58] . H3 tri-methyl lysine 36 (αH3K36me3) (Abcam 9050), H3 di-methy lysine 36 (αH3K36me2) (Abcam 9049), H3 mono-methyl lysine 36 (αH3K36me1) (Abcam 9048) and H3 lysine 36 acetylation (Active Motif 39379) were used at a dilution of 1:1,000. An antibody directed against H3 (Abcam1791) was used as a loading control. Anti-rabbit horseradish peroxidase-conjugated secondary antibodies (Amersham Bioscience) were used at a dilution of 1:10,000. For clarity, western blots were cropped to show the band of interest in the main figures. However, corresponding uncropped scans can be found in Supplementary Fig. 10 and Supplementary Fig. 11 . Accession codes: The microarray data have been deposited with ArrayExpress ( https://www.ebi.ac.uk/arrayexpress/ ) under accession code E-MTAB-2549 . How to cite this article: Pai, C.-C. et al. A histone H3K36 chromatin switch coordinates DNA double-strand break repair pathway choice. Nat. Commun. 5:4091 doi: 10.1038/ncomms5091 (2014).